TEMPRANILLOgenes link photoperiod and gibberellin pathways to control flowering inArabidopsis In Arabidopsis , FLOWERING LOCUS T ( FT ) promotes flowering in response to long days in the photoperiod pathway, while signalling downstream gibberellin (GA) perception is critical for flowering under short days. Previously we have established that the TEMPRANILLO ( TEM ) genes have a pivotal role in the direct repression of FT . Here we show that TEM genes directly regulate the expression of the GA 4 biosynthetic genes GA 3–oxidase1 and 2 ( GA3OX1 and GA3OX2 ). Plants overexpressing TEM genes resemble GA-deficient mutants, and conversely, TEM downregulation give rise to elongated hypocotyls perhaps as a result of an increase in GA content. We consistently find that TEM1 represses GA3OX1 and GA3OX2 by directly binding a regulatory region positioned in the first exon. Our results indicate that TEM genes seem to link the photoperiod and GA-dependent flowering pathways, controlling floral transition under inductive and non-inductive day lengths through the regulation of the floral integrators. In plants, flowering is controlled by different genetic pathways that monitor the developmental stage as well as the environmental conditions. In Arabidopsis , the convergence of flowering pathways results in the activation of the floral pathway integrators, FLOWERING LOCUS T ( FT ) and SUPPRESSOR OF OVEREXPRESSOR OF CO 1 ( SOC1 ), which in turn activate the floral meristem identity genes in the shoot apical meristem (SAM) [1] , [2] . In the photoperiod pathway, FT promotes flowering in response to increasing long days (LD). We have previously found that the TEMPRANILLO (TEM) genes have a pivotal role in the direct repression of FT and counteract the activator CONSTANS ( CO ) [3] . A quantitative balance between TEM and CO, both regulated by light and the circadian clock, controls FT accumulation in LD [3] . In addition, it has recently been suggested that GIGANTEA, an output from the circadian clock, directly regulates FT expression through neutralization of TEM (1 and 2) and SHORT VEGETATIVE PHASE [4] , two FT repressors [3] , [5] , [6] . Here, we show that TEM1 and TEM2 act redundantly in the photoperiod pathway repressing floral induction. In addition, results from the short days (SD)–LD shift experiment suggest that TEM genes are differentially expressed in SD and LD, and their prompt downregulation upon day-time extension may account for the upregulation of FT in increasing day length. Under SD, signalling downstream gibberellin (GA) perception is critical for flowering [7] , as GA accumulation induces SOC1 and LEAFY ( LFY) expression in the SAM [8] , [9] . However, the mechanism responsible for the rise in GA levels that ultimately triggers flowering under SD is largely unknown. We demonstrate that TEM gene products are direct repressors of two related genes that encode enzymes able to catalyse the last step of GA biosynthesis. TEM1 and TEM2 repress flowering under LD and SD conditions Flowering time of tem mutants is also affected in SD ( Fig. 1 ), better observed with the isolation of a novel loss of function tem2 allele ( tem2-2 , Supplementary Fig. S1 ), which enhanced the early flowering phenotype of the tem1-1 mutant under both LD and SD conditions ( Fig. 1 ). Under LD, tem1-1 and tem2-2 single mutants flowered earlier than wild-type plants, and tem1-1 tem2-2 double mutants flowered much earlier than single mutants but similarly to CO overexpressor ( 35S :: CO ) plants ( Fig. 1a–c ). FT expression was increased from day 8 in tem1-1 and tem2-2 , whereas in the double mutant its transcript levels were already high on day 6 ( Fig. 1d ), when plants had only formed the first two true leaves. At bolting, 35S :: CO and tem1-1 tem2-2 plants had formed five rosette leaves whereas the wild type developed about ten leaves ( Fig. 1b ). Under SD, CO overexpressors flowered at the same time as in LD [10] , [11] , but tem1-1 tem2-2 double mutants flowered after producing ten rosette leaves, much earlier than wild-type plants although slightly later than in LD ( Fig. 1e,f ). These results confirmed that TEM1 and TEM2 act redundantly to repress FT in LD and suggested that may also have a role in SD. 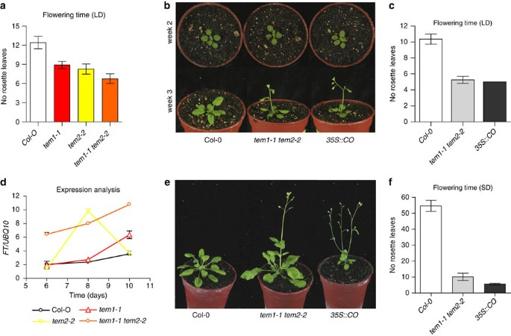Figure 1: Early flowering phenotype oftem1-1 tem2-2double mutants under LD and SD. (a) Flowering time of single and doubletem1-1 tem2-2mutants under LD. (b) Wild-type, double mutant and35S::COplants after 2 and 3 weeks growth under LD. (c) Flowering time of double mutant and35S::COplants compared with the wild type under LD. (d) RT–qPCR analysis ofFTexpression at ZT16 in single and doubletem1-1 tem2-2mutants grown in LD. The two biological replicates gave the same results, and one was chosen as representative with error bars of three technical replicates. (e) Wild-type, double-mutant and35S::COplants grown 6 weeks under SD. (f) Flowering time of double-mutant and35S::COplants compared with the wild type SD. Error bars indicate s.d. of the mean number of rosette leaves of 20 plants for each genotype. Figure 1: Early flowering phenotype of tem1-1 tem2-2 double mutants under LD and SD. ( a ) Flowering time of single and double tem1-1 tem2-2 mutants under LD. ( b ) Wild-type, double mutant and 35S :: CO plants after 2 and 3 weeks growth under LD. ( c ) Flowering time of double mutant and 35S :: CO plants compared with the wild type under LD. ( d ) RT–qPCR analysis of FT expression at ZT16 in single and double tem1-1 tem2-2 mutants grown in LD. The two biological replicates gave the same results, and one was chosen as representative with error bars of three technical replicates. ( e ) Wild-type, double-mutant and 35S :: CO plants grown 6 weeks under SD. ( f ) Flowering time of double-mutant and 35S :: CO plants compared with the wild type SD. Error bars indicate s.d. of the mean number of rosette leaves of 20 plants for each genotype. Full size image TEM genes are differentially expressed under LD and SD Changes in TEM diurnal cycling in response to photoperiod were then monitored. Under SD, TEM messenger RNA (mRNA) levels were low during the day, started to increase at dusk and peaked at ZT12 (ZT stands for Zeiteberg Time or hours after lights were switched on) in wild-type seedlings. TEM1 and TEM2 expression patterns were similar, but TEM2 had a smaller peak late at night ( Fig. 2a ). To further investigate the effect of day length on the regulation of TEM genes, we performed a SD–LD shift experiment. Light in the subjective night of SD-entrained wild-type plants affected their oscillation pattern immediately after the shift ( Fig. 2a ). As soon as plants were transferred to LD, the peak of TEM1 expression was displaced from ZT12 to ZT18 (typical of LD) with an almost 50% decrease in amplitude at least in the first two LDs. TEM2 showed two peaks of expression at ZT12 and ZT24 in control plants, but the first peak disappeared in plants exposed to LD. As has been previously demonstrated [12] , FT mRNA expression remained low in plants grown under SD, whereas there was a significant increase in plants shifted to LD ( Fig. 2a ). When shifted back to SD, the peaks of expression of TEM genes were re-established and FT transcription fell to very low levels ( Fig. 2a ). Therefore, TEM gene expressions responded rapidly to photoperiod switches, which resulted in changes in FT expression. Similarly, through immunodetection using a TEM1-specific antibody on protein extracts from wild-type seedlings, we found that TEM1 protein accumulation mirrored the pattern of TEM1 mRNA expression. Under LD, it accumulates in the late afternoon and reaches the highest levels at night ( Fig. 2b ). Also, higher protein accumulation and at earlier ZT times was observed in SD related to higher mRNA expression levels in these conditions ( Fig. 2c ). 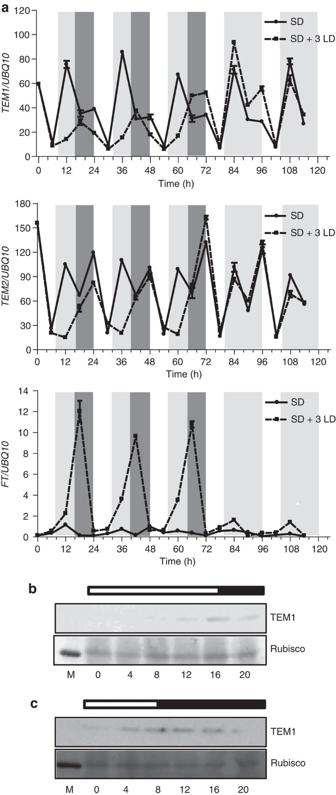Figure 2: Accumulation ofTEMmRNA and protein in response to photoperiod. (a) SD–LD shift. Wild-type seedlings were entrained for 2 weeks under SD; on day 15, half the plants were moved to LD for 3 days and then returned to SD, whereas half the plants remained under SD as control. Samples were collected every 6 h for 5 days for RT–qPCR analysis. Relative mRNA levels ofTEM1(top panel),TEM2(middle panel) andFT(bottom panel) in control plants grown under SD (solid line) and in plants exposed to 3 LD (dotted line). In light grey, 16-h night (SD); in dark grey, 8-h night (LD). The two biological replicates gave the same results; one was chosen as representative, shown with error bars of three qPCR replicates. (b,c) Diurnal accumulation of TEM1 protein in wild-type seedlings grown under LD and SD, respectively. For immunodetection, 20 seedlings for each time point were collected every 4 h from ZT0 to ZT20. As loading control, Rubisco was visible after Red Ponceau staining. Three biological replicates gave similar results, and one was chosen as representative. M, marker. Figure 2: Accumulation of TEM mRNA and protein in response to photoperiod. ( a ) SD–LD shift. Wild-type seedlings were entrained for 2 weeks under SD; on day 15, half the plants were moved to LD for 3 days and then returned to SD, whereas half the plants remained under SD as control. Samples were collected every 6 h for 5 days for RT–qPCR analysis. Relative mRNA levels of TEM1 (top panel), TEM2 (middle panel) and FT (bottom panel) in control plants grown under SD (solid line) and in plants exposed to 3 LD (dotted line). In light grey, 16-h night (SD); in dark grey, 8-h night (LD). The two biological replicates gave the same results; one was chosen as representative, shown with error bars of three qPCR replicates. ( b , c ) Diurnal accumulation of TEM1 protein in wild-type seedlings grown under LD and SD, respectively. For immunodetection, 20 seedlings for each time point were collected every 4 h from ZT0 to ZT20. As loading control, Rubisco was visible after Red Ponceau staining. Three biological replicates gave similar results, and one was chosen as representative. M, marker. Full size image TEM silencing affects flowering and hypocotyl elongation It has been proposed that TEM acts in leaves, together with CO, to tightly control FT accumulation [3] ; however, TEM expression is also detected, by in situ hybridization and β-glucuronidase (GUS) staining, in the SAM and the hypocotyl ( Supplementary Fig.S2a,b ). Therefore, we expressed an artificial miRNA targeted against both TEM genes under the control of the KNAT1 promoter to drive their silencing in the SAM [13] , [14] ( Supplementary Fig. S2c ). As a control, we employed the 35S promoter to test the effectiveness of the silencing ( p35S :: amiR-TEM ). We detected downregulation of both TEM genes in whole plants and in SAM- and hypocotyls-enriched tissue of pKNAT1 :: amiR-TEM lines and in p35S :: amiR-TEM whole plants ( Supplementary Fig. S2d–f ). This downregulation was directly associated to the upregulation of FT expression ( Supplementary Fig. S2d,f ) and to the early flowering phenotype in LD ( Fig. 3a , Supplementary Fig. S2g ), which strongly suggested that TEM also had a role in controlling flowering in the SAM. 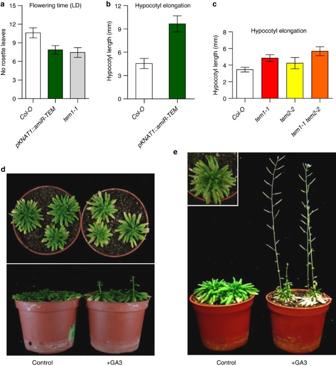Figure 3: GA-related phenotypes ofTEMmisexpression. (a) Flowering time ofpKNAT1:amiR-TEMT3lines under LD. Error bars are the s.d. of the mean number of rosette leaves of 30 plants of each line. (b,c) Hypocotyl elongation in SD-grown seedlings ofpKNAT1:amiR-TEMand single and doubletemmutants compared with the wild type, respectively. The length of hypocotyls is reported as the mean value with s.e. of 20 seedlings for each genotype. (d,e)35S::TEM1plants treated with 100 μM GA3(right) compared with untreated plants (left) grown under SD for 12 (d) and 20 weeks (e). In the close-up,35S:TEM1plants in the vegetative phase. The two biological replicates gave similar results. Figure 3: GA-related phenotypes of TEM misexpression. ( a ) Flowering time of pKNAT1:amiR-TEM T 3 lines under LD. Error bars are the s.d. of the mean number of rosette leaves of 30 plants of each line. ( b , c ) Hypocotyl elongation in SD-grown seedlings of pKNAT1:amiR-TEM and single and double tem mutants compared with the wild type, respectively. The length of hypocotyls is reported as the mean value with s.e. of 20 seedlings for each genotype. ( d , e ) 35S :: TEM1 plants treated with 100 μM GA 3 (right) compared with untreated plants (left) grown under SD for 12 ( d ) and 20 weeks ( e ). In the close-up, 35S:TEM1 plants in the vegetative phase. The two biological replicates gave similar results. Full size image Moreover, we observed that these pKNAT1 :: amiR-TEM plants had elongated hypocotyls ( Fig. 3b ). When we analysed SD-grown seedlings, we also found the hypocotyl phenotype in p35S :: amiR-TEM and tem mutant plants ( Supplementary Fig. 3a , Fig. 3c ). This meant that lines in which TEM genes were silenced at least in the hypocotyl and SAM [15] , [16] had elongated hypocotyls both in LD and SD ( Fig. 3b , Supplementary Fig. S3b–d ), while plants overexpressing TEM genes had a dwarf phenotype, loss of apical dominance, extremely late flowering ( Supplementary Fig. S4a,b ) and shorter hypocotyls (see Fig. 4c ). The fact that all these phenotypes might be related to unbalanced GA levels [17] , [18] prompted us to study the interplay of TEM genes and the GA pathway, which has been proposed to have a major role in inducing flowering in SD [7] , [19] . 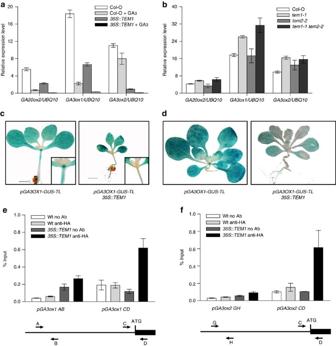Figure 4: TEM regulates GA biosynthetic genes. (a,b) Expression analysis of GA metabolism genes in wild-type and35S::TEM1seedlings, and in wild-type,tem1-1,tem2-2andtem1-1 tem2-2mutants. After 1 week under SD, samples were collected at ZT8 and subjected to RT–qPCR. (c,d) GUS staining ofpGA3OX1-GUS-TLandpGA3OX1-GUS-TL 35S::TEM1(F3) grown for 10 days under SD (SAM close-up in the inset) and for 3 weeks under LD. Bar represents 1 cm. (e) ChIP analysis of TEM1 binding toGA3OX1regulatory regions. Precipitated chromatin was used as template in qPCR with primer sets AB, amplifying a region 2.4 kb upstream of the ATG, and CD, amplifying the region of the first exon containing the RAV-binding site. (f) ChIP analysis of TEM1 binding toGA3OX2regulatory regions. Precipitated chromatin was used as template in qPCR with primer sets GH, amplifying a region 2.7 kb upstream of the ATG, and CD, amplifying the region of the first exon containing a non-canonical RAV-binding site. For expression and ChIP analyses, three biological replicates were performed with similar results. One representative is shown with error bars of three qPCR replicates; other biological replicates are shown inSupplementary Fig. S6b. Wt, wild type. Figure 4: TEM regulates GA biosynthetic genes. ( a , b ) Expression analysis of GA metabolism genes in wild-type and 35S :: TEM1 seedlings, and in wild-type, tem1-1 , tem2-2 and tem1-1 tem2-2 mutants. After 1 week under SD, samples were collected at ZT8 and subjected to RT–qPCR. ( c , d ) GUS staining of pGA3OX1-GUS-TL and pGA3OX1-GUS-TL 35S :: TEM1 (F3) grown for 10 days under SD (SAM close-up in the inset) and for 3 weeks under LD. Bar represents 1 cm. ( e ) ChIP analysis of TEM1 binding to GA3OX1 regulatory regions. Precipitated chromatin was used as template in qPCR with primer sets AB, amplifying a region 2.4 kb upstream of the ATG, and CD, amplifying the region of the first exon containing the RAV-binding site. ( f ) ChIP analysis of TEM1 binding to GA3OX2 regulatory regions. Precipitated chromatin was used as template in qPCR with primer sets GH, amplifying a region 2.7 kb upstream of the ATG, and CD, amplifying the region of the first exon containing a non-canonical RAV-binding site. For expression and ChIP analyses, three biological replicates were performed with similar results. One representative is shown with error bars of three qPCR replicates; other biological replicates are shown in Supplementary Fig. S6b . Wt, wild type. Full size image GA metabolism genes are altered in TEM misexpressing lines First, 35S :: TEM1 plants were treated with 100 μM GA 3 to determine whether exogenous GA could rescue their late flowering phenotype in SD. In 35S :: TEM1 plants treated with GA 3 , bolting was evident from week 12 similarly to untreated SD-grown wild types that bolt from week 10 ( Fig. 3d , Supplementary Fig. S4c , Supplementary Table S1 ). In contrast, only a few untreated 35S :: TEM1 plants flowered after 5 months under SD, and most of them remained in the vegetative phase, producing leaves indefinitely ( Fig. 3e , Supplementary Table S1 ). The rescue of the apical dominance and flowering phenotypes obtained with GA treatment ( Fig. 3d,e ) suggested that TEM genes could be involved in the GA pathway. We analysed the expression of GA metabolism genes [20] , [21] , [22] in wild-type and 35S :: TEM1 seedlings grown under SD in basic medium or medium supplemented with 10 μM GA 3 . We confirmed that GA metabolic genes are subjected to complex regulation based on negative feed-back and positive feed-forward mechanisms (reviewed in ref. 23 ) owing to an excess of GA in the growth medium in both genotypes ( Fig. 4a , Supplementary Fig. S5a ). In addition, there was a significant downregulation of GA 20–oxidase2 ( GA20OX2 ), GA3OX1 and GA3OX2 in TEM1 overexpressors compared with the wild type ( Fig. 4a ), indicating a possible involvement of TEM in the regulation of GA biosynthesis genes. We then monitored the expression of these genes in tem single- and double-mutant seedlings, and found that GA3OX1 and GA3OX2 were significantly upregulated in tem1-1 and tem1-1 tem2-2 ( Fig. 4b ) indicating that these two GA3OX genes are repressed by TEM. In addition, at least GA3OX1 also displayed a clear diurnal oscillation, with a peak of expression at ZT8 in SD ( Supplementary Fig. S5b ). This finding is consistent with the decrease of GA3OX1 expression at ZT12, the time at which TEM levels peak. To further support the downregulation of GA3OX1 by TEM, 35S:: TEM1 [3] plants were crossed with a reporter line in which β-glucuronidase expression is driven by the GA3OX1 promoter and first exon [20] . In young 35S :: TEM1 pGA3OX1-GUS-TL plants, GUS staining was visible in cotyledons but not in the SAM, whereas in older plants we observed a general downregulation of GUS expression also in leaves ( Fig. 4c,d ). The GA3–oxidase1 downregulation should ensure reduced GA content [20] . GA3OX1 and GA3OX2 are novel direct targets of TEM1 As previously reported, TEM specifically binds a sequence known as the RAV1 recognition site [3] , [24] ( Supplementary Table S2a ). We identified this sequence in the promoter region of the AtGID1c gene, encoding a GA receptor, and in the first exon of the GA3OX1 gene ( Supplementary Table S2b,c ). The direct binding of TEM1 to putative targets was then assayed by chromatin immunoprecipitation (ChIP) using the 35S :: TEM1 line [3] . No enrichment was found for pGID1c ( Supplementary Fig. S6a ), but there was significant enrichment in a region containing the RAV-binding site at the first exon of GA3OX1 , but not in a region 2.4 kb upstream of the ATG ( Fig. 4e ). In addition, we found a significant enrichment in the same region of the first exon of GA3OX2 , containing a non-canonical RAV-binding site ( Supplementary Table S6d ), but not in a region 2.7 kb upstream of the ATG ( Fig. 4f ). These data indicated that TEM1 directly binds and regulates the expression of the GA 4 biosynthetic genes GA3OX1 and GA3OX2 . In SD, flowering is mainly promoted by the plant hormones GAs through the activation of the floral integrator SOC1 [8] and the floral meristem identity gene LFY in the apical meristem [19] , although they also seem to have a role in LD [20] , [25] , [26] . We found that ga3ox1 mutation delays the early flowering of tem1 tem2 double mutants, as in LD tem1-1 tem2-2 plants generated 6.53±0.80 rosette leaves whereas tem1 tem2 ga3ox1 triple mutant plants flowered after producing 8.09±0.66 rosette leaves ( Table 1 ). This corroborated that at least a part of the TEM role in flowering is through the regulation of GA3OX1 . Table 1 Number of rosette leaves before bolting under LD. Full size table SOC1 and LFY are upregulated in tem mutants under LD and SD As mentioned previously, GAs promote flowering through the activation of SOC1 and LFY both in LD and SD [19] , [20] , [25] , [26] , therefore we compared the expression levels of these positive floral activators in wild-type and tem1-1 tem2-2 mutant plants grown under SD and LD before their respective wild-type floral induction times. At all time points tested, SOC1 and LFY, as well as GA3OX1 , were upregulated in the tem1-1 tem2-2 double mutant with a 2–3 fold increase ( Fig. 5a,b , Supplementary Fig. S7 ). GA3OX2 gene was also upregulated in tem double mutants at the earlier time point, but to a lesser extent ( Fig. 5a,b , Supplementary Fig. 7 ). 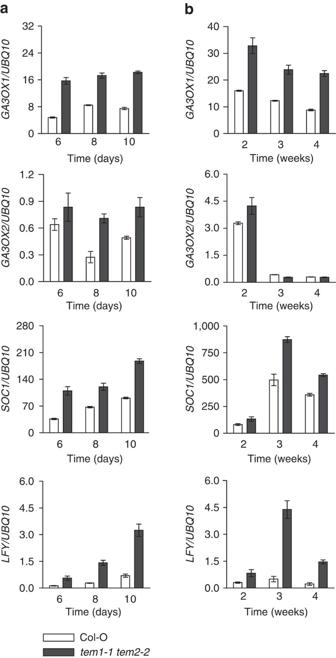Figure 5: De-repression ofSOC1,LFY, and GA biosynthetic genes intemdouble mutants. Expression analysis ofGA3OX1, GA3OX2,SOC1andLFYgenes in wild-type andtem1-1 tem2-2mutant grown under LD (a) and SD (b) before flowering. Pools of ten plants for each time point were collected at ZT12 at day 6, 8 and 10 under LD and at ZT8 at week 2, 3 and 4 under SD. Two biological replicates gave similar results, one representative is shown with error bars of three qPCR replicates. Several other biological replicates are shown inSupplementary Fig. S7. Figure 5: De-repression of SOC1 , LFY , and GA biosynthetic genes in tem double mutants. Expression analysis of GA3OX1, GA3OX2 , SOC1 and LFY genes in wild-type and tem1-1 tem2-2 mutant grown under LD ( a ) and SD ( b ) before flowering. Pools of ten plants for each time point were collected at ZT12 at day 6, 8 and 10 under LD and at ZT8 at week 2, 3 and 4 under SD. Two biological replicates gave similar results, one representative is shown with error bars of three qPCR replicates. Several other biological replicates are shown in Supplementary Fig. S7 . Full size image Our new data using the novel allele tem2-2 confirmed that TEM1 and TEM2 act redundantly to repress FT in LD, therefore delaying flowering. Consequently, plants lacking the FT repressors resembled plants in which the activator of FT is constitutively expressed ( Fig. 1b,c ). Moreover, tem double mutants still responded to changes in the photoperiod, and their early flowering phenotype under SD indicated an additional role of TEM in SD conditions. Plants grown under SD are late flowering; however, they flower earlier if exposed to three LDs due to transient upregulation of FT in the leaf [12] . The shift experiment confirmed that TEM genes are differentially expressed in SD and LD, and showed that they are immediately downregulated on day-length extension ( Fig. 2a ). Therefore, we propose that the loss of the ZT12 peak of TEM contributes to the sharp upregulation of FT in LD. Under SD conditions, plants flower in response to the GA pathway as endogenous accumulation of the phytohormone GA induces SOC1 and LFY expression in the SAM [7] . Mutants defective in the biosynthesis of GA exhibit dramatic delays in the timing of flowering particularly when grown under SD, suggesting that GA is an important stimulator of flowering in the absence of an active LD promotion pathway [8] , [19] . The fact that plants overexpressing TEM genes resembled GA-deficient mutants, and that conversely, TEM downregulation gave rise to elongated hypocotyls perhaps as a result of an increase in GA content, suggested a link of TEM with the GA pathway. GA 3 treatment rescued the plant apical dominancy and accelerated flowering of 35S :: TEM1 plants indicating that TEM1 may control genes of the GA pathway. However, the fact that GA 3 -treated 35S :: TEM1 plants flowered later than wild-type-treated plants suggested that TEM may have among its targets other genes unrelated to the GA pathway. We consistently found that TEM1 directly represses GA3OX1 and GA3OX2 , and that these genes were upregulated in tem1 single and tem1 tem2 double mutants, suggesting a major effect of TEM1 on GA3OX gene regulation and a link between TEM and genes encoding enzymes that catalyse the last step of GA 4 biosynthesis. Moreover, GA3OX1 displayed diurnal oscillation and its decrease of expression at ZT12 under SD ( supplementary Fig. S5b ) correlates with the peak of expression of TEM ( Fig. 2a ). The direct repression of GA3OX genes would result in a reduction of bioactive GA 4 , as it has been shown that in the single ga3ox1-3 mutant the level of bioactive GA 4 decreases and in the double ga3ox1 ga3ox2 mutant the amount of GA 4 is almost undetectable, which correlates with their late flowering phenotypes [20] . Therefore, the early flowering phenotype of tem1 tem2 double mutants may be at least in part due to the GA3–oxidase1 upregulation as ga3ox1 mutation delays the tem1 tem2 precocious flowering. The fact that triple tem1 tem2 ga3ox1 mutant plants flowered earlier than ga3ox1 single mutants and similarly to wild types ( Table 1 ) would likely be due to the FT upregulation in the tem double-mutant background ( Fig. 1d ). The upregulation of GA3–oxidase genes in tem mutant backgrounds is likely the result of the absence of the repressor TEM and of the action of an unidentified GA3OX activator. In addition, the activation of SOC1 and LFY at early stages of development in double-mutant plants would be likely due to the higher content of the bioactive GA 4 as a consequence of both GA3OX upregulation ( Fig. 5 ) and higher levels of FT expression ( Fig. 1d ). In conclusion, our data indicate that TEM downregulation is required in order to get enough FT and GA3OX1 and GA3OX2 expression to induce flowering. Therefore, TEM links both pathways by directly repressing FT and GA3OX genes, which are responsible for the production of the mobile signals that induce flowering at SAM. Consequently, it seems to have a critical role in leaves and SAM, and both in LD and SD. We anticipate this to be a general mechanism to avoid precocious flowering. As previously suggested, the GA pathway is also active in LD [27] but its action is masked by the photoperiod pathway; however, it becomes evident in co and ft mutants or in SD. It has already been shown that the GA pathway seems to be controlled by photoperiod [28] , [29] , and we propose that the GA signalling pathway might be controlled by day length via direct binding of TEM to two related genes involved in the production of bioactive GA 4 . Plant material and growth conditions Seeds were stratified for 3 days at 4 °C, and plants were grown in controlled conditions at 22 °C, under LD (16 h light/8 h dark) or SD (8 h light/16 h dark). Transgenic lines are reported in Supplementary Table S3 . GA treatment was performed as previously described in ref. 8 . A total of 50 plants (wild-type and 35S:TEM1 ) were grown under SD, and half were sprayed with 100 μM GA 3 twice a week, from week 2 to week 8. Cloning The amiRNA sequence targeted against TEM genes was amplified by PCR according to Schwab et al . [30] . For constitutive silencing, amiR-TEM was cloned as a Sal I– Bam HI fragment in pBIN-JIT. For tissue-specific silencing, the amiR-TEM was cloned as a Kpn I- Not I restriction fragment in a modified Gateway entry vector in which the KNAT1 promoter and the Nos terminator were previously cloned. The Nos terminator was amplified by PCR, and cloned in pENTR-3C as a Kpn I– EcoR V restriction fragment. The KNAT1 promoter was amplified by PCR, and cloned in pENTR3C-Nos terminator as a Sal I– Bam HI fragment. The pENTR plasmid containing pKNAT1 :: amiR-TEM was linearized with NheI, dephosphorylated with alkaline phosphatase and recombined by the LR reaction into MDC123, a Gateway-compatible binary vector described by Curtis and Grossniklaus [31] . For PCR reactions, Col-O genomic DNA was used as template with specific primers as listed in Supplementary Table S4 . All PCR products were subcloned in pCRII and verified by sequencing. Agrobacterium tumefaciens (PGV2260 strain) was electroporated with plant expression vectors, and used to transform wild-type plants by floral dip. At least 5–10 T 1 transgenic lines for each construct were selected on MS1 supplemented with the appropriate antibiotic. Phenotypic analyses For hypocotyls elongation, 5-DAG seedlings were laid horizontally and digital pictures were taken. Hypocotyl length was measured using a standard 10-mm ruler with Image J software. For flowering time, all the experiments were performed on soil-grown plants at least twice. Data are reported as mean value of the number of rosette leaves of 20–30 plants, each genotype with s.d. Expression analysis pTEM1 :: GUS seedlings were used for GUS expression analyses [3] . GUS staining was as described elsewhere [32] . In situ hybridization was as previously described [33] . TEM1 probe was generated from pCC54 plasmid containing a TEM1 296-bp HincII fragment. For quantitative reverse transcription PCR (RT–qPCR) reactions, seeds were surface sterilized and seedlings were grown under controlled conditions on MS1, with the exception of expression analysis throughout development for which plants were grown on soil. RNA was extracted from a pool of 20 seedlings (whole seedlings or seedlings with excised cotyledons resulting in hypocotyls-/SAM-enriched tissues) or 10 adult plants with PureLink RNA Mini Kit (Ambion), treated with DNaseI RNase free (Ambion), and 1 μg was retrotranscribed with oligo(dT) and SuperScript III (Invitrogen). The expression levels of genes of interest were monitored by qPCR using SYBR Green I Master Mix and Light Cycler 480 (Roche) with the primers as listed in Supplementary Table S5 . Data were normalized using the UBQ10 gene as reference. For GA metabolism genes, we chose to study only those genes that encode enzymes involved in the final steps of GA biosynthesis, that are highly expressed during the vegetative phase and for which mutants have already been described in the literature as affected in their flowering time phenotype [21] , [22] . AtGA20OX2 , AtGA3OX1 and 2 encode enzymes responsible for the conversion of GA precursors to bioactive forms, whereas AtGA2OX2 and 4 encode enzymes responsible for the catabolism of bioactive GAs. TEM1 protein accumulation To determine TEM1 protein accumulation, specific antibodies were raised against a TEM1 synthetic peptide (from aa 18 to aa 31, ISTTPKPTTTTEKK) and first tested in dot-blot experiments. α-TEM1 was able to recognize GST-TEM1 recombinant protein only in denatured samples (not shown), so could only be used in immunodetection in denatured samples, not for in vivo assays (co-immunoprecipitation and ChIP). For time-course experiments, 20 seedlings for each time point (1-week-old grown under LD and 2-weeks-old grown under SD) were collected and ground in liquid nitrogen. Proteins were extracted in RIPA buffer (50 mM Tris–HCl pH 8.0, 150 mM NaCl, 1% NP-40, 0.1% SDS, 0.5% sodium deoxycholate, 0.5% polyvinylpolypyrrolidone, 1 mM phenylmethylsulphonyl fluoride, 5 mg ml −1 leupeptin, 1 mg ml −1 aprotinin, 5 mg ml −1 antipain and 1 mg ml −1 pepstatin) and their concentration was calculated using the Bradford method (Bio-Rad) in a Spectramax microplate reader. For western blot, 20 μg of total protein extract was loaded per lane. After SDS–PAGE, separated proteins were transferred to nitrocellulose membranes (Protran and Whatmann) and stained with Ponceau Red. The presence of TEM1 protein was detected using a rabbit primary antibody raised against a synthetic peptide (both produced by Abyntek), and a secondary peroxidase-conjugated goat anti-rabbit antibody (Pierce). Chemiluminescence was performed using the SuperSignal West Femto Maximum sensitivity substrate (Pierce), and protein accumulation was quantified using the LAS-4000 imaging system (Fujifilm–GE Healthcare). Chromatin immunoprecipitation The direct binding of TEM1 to putative targets was assayed using the 35S :: TEM1 line as previously described [3] . The crosslinked DNA was immunoprecipitated with an anti-HA antibody (Sigma), purified using Protein A-Agarose resin (Millipore) and tested by qPCR using different primer sets spanning regulatory regions of putative direct targets (as listed in Supplementary Table S6 ). How to cite this article: Osnato, M. et al . TEMPRANILLO genes link photoperiod and gibberellin pathways to control flowering in Arabidopsis . Nat. Commun. 3:808 doi: 10.1038/ncomms1810 (2012).